Temporal tweezing of light through the trapping and manipulation of temporal cavity solitons Optical tweezers use laser light to trap and move microscopic particles in space. Here we demonstrate a similar control over ultrashort light pulses, but in time. Our experiment involves temporal cavity solitons that are stored in a passive loop of optical fibre pumped by a continuous wave ‘holding’ laser beam. The cavity solitons are trapped into specific time slots through a phase modulation of the holding beam, and moved around in time by manipulating the phase profile. We report both continuous and discrete manipulations of the temporal positions of picosecond light pulses, with the ability to simultaneously and independently control several pulses within a train. We also study the transient drifting dynamics and show complete agreement with theoretical predictions. Our study demonstrates how the unique particle-like characteristics of cavity solitons can be leveraged to achieve unprecedented control over light. These results could have significant ramifications for optical information processing. All-optical trapping and manipulation of the temporal positions of light pulses is a highly desirable functionality, with immediate ramifications for optical information processing [1] , [2] , [3] , [4] . Information represented as a sequence of pulses could be stored and reconfigured on the fly, without the need for power-hungry optoelectronic conversion. This calls for the ability to trap ultrashort pulses of light, and dynamically move them around in time, with respect to, and independently of each other. Slow-light [5] , [6] , [7] , [8] , [9] and nonlinear cross-phase modulation effects [10] , [11] , [12] , [13] , [14] can partly achieve this feat, yet neither of these approaches are sufficiently flexible to enable independent dynamical control of light pulses within a sequence. Enter temporal cavity solitons (CSs) [15] , [16] , [17] , [18] , [19] , [20] . These are the dissipative solitons [21] , [22] of externally driven nonlinear passive cavities. Specifically, they are pulses of light that can persist indefinitely in a passive loop of nonlinear optical material such as fibre rings [16] , [17] , [18] , [19] and monolithic microresonators [20] , without changing shape or losing power. Dispersive temporal spreading is arrested by the material nonlinearity, and they draw the power they need from a continuous wave (cw) ‘holding’ laser beam driving the cavity. As multiple CSs can be present simultaneously and independently, at arbitrary temporal positions, they constitute ideal bits for all-optical buffer applications [16] . Furthermore, their ‘plasticity’ provides a solution to the problem of selective positioning control. Specifically, any gradient on the cavity holding beam is expected to cause an overlapping CS to move towards—and be trapped at—a point where the gradient vanishes. Dynamical control of these external gradients then shifts the CSs. This concept has been investigated theoretically in the context of two-dimensional spatial CSs, beams of light persisting in the transverse plane of planar cavities [1] , [2] , [23] , [24] , [25] , [26] , [27] . Although experiments have had some success in positioning and moving spatial CSs in space, local defects and non-uniformities across the plane of the cavity often somewhat restrict this control [8] , [28] , [29] , [30] , [31] , [32] , [33] . With temporal CSs, material imperfections are not an issue: every CS circulating in the cavity sees the same averaged environment [34] . Integration with existing fibre-optic communication technologies is also more natural. Here we report on the experimental realization of trapping and selective manipulation of temporal cavity solitons. In our experiment, the CSs exist as picosecond pulses of light, recirculating in a loop of optical fibre, and we expose them to temporal control gradients in the form of a gigahertz phase modulation imposed on the cavity holding beam. We show theoretically and experimentally that CSs are attracted and trapped to phase maxima, effectively suppressing environmental fluctuations, as well as acoustic interactions [18] that otherwise would play a role not dissimilar to material defects. By dynamically changing the phase pattern, we then controllably move the CSs in time, in essence selectively speeding them up or slowing them down. Continuous and discrete manipulations are demonstrated, both with temporal shifts much larger than the CS duration. In addition, we investigate the transient CS attraction dynamics, and show complete agreement with theoretical predictions. Our results demonstrate that individual ultrashort light pulses can be shifted temporally, forward or backward, simply using cw laser light. This compares with conventional optical tweezers that trap and move microscopic particles in space [35] , [36] , [37] , only here we manipulate light itself, and in time. We therefore refer to our technique as the temporal tweezing of light. 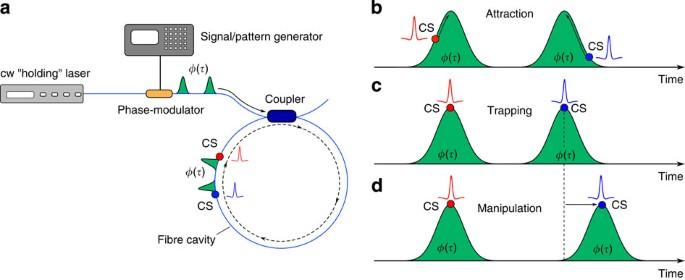Figure 1: Principle of the temporal tweezing of light. (a) A cw laser with an imprinted phase patternφ(τ) (green) drives a passive fibre cavity. (b) When optical temporal CSs (red and blue) circling the cavity overlap with a phase gradient, their velocity changes and they drift towards the nearest phase maxima. (c) The maxima act as temporal trapping sites for the CSs. (d) Once trapped, the CSs follow changes in the phase pattern: modifying the relative delay of two phase maxima enables arbitrary manipulation of the temporal delay of two CSs. Concept of temporal tweezing Figure 1 illustrates the principle underlying temporal tweezing. We consider a passive resonator constructed of single-mode optical fibre, driven with monochromatic laser light. A modulator imprints a time-varying electric signal φ ( τ ) onto the phase of the cw holding laser driving the cavity. Provided that φ ( τ ) repeats periodically, with a period that is an integer fraction of the cavity roundtrip time, the holding beam builds up over several roundtrips an intracavity cw field with an identical travelling phase pattern ( Supplementary Note 1 ). Being effectively synchronized to the phase modulation, the intracavity phase pattern is coherently reinforced each roundtrip, ensuring steady-state operation. Figure 1: Principle of the temporal tweezing of light. ( a ) A cw laser with an imprinted phase pattern φ ( τ ) (green) drives a passive fibre cavity. ( b ) When optical temporal CSs (red and blue) circling the cavity overlap with a phase gradient, their velocity changes and they drift towards the nearest phase maxima. ( c ) The maxima act as temporal trapping sites for the CSs. ( d ) Once trapped, the CSs follow changes in the phase pattern: modifying the relative delay of two phase maxima enables arbitrary manipulation of the temporal delay of two CSs. Full size image Temporal CSs circulating around the cavity are superimposed onto the cw intracavity field. They normally have the same frequency and group velocity as that field [16] . However, the presence of a phase gradient across a light pulse is equivalent to an instantaneous frequency shift, δ ω =−d φ /d τ =− φ ′. Specifically, a decrease (respectively, increase) of phase over time leads to a blue-shift (red-shift). In a material exhibiting anomalous dispersion (a necessary condition for temporal CSs to exist [16] ), this shift translates into an increase (respectively, decrease) of the group velocity. Accordingly, the temporal CSs catch up with the imprinted phase pattern (or vice versa), leading to an effective time-domain drift of the CSs towards the nearest phase maxima. Over one roundtrip, the CSs accrue an extra group delay given by (see also Supplementary Note 1 ): where L is the length of the fibre loop and β 2 is the group velocity dispersion coefficient, and we have assumed anomalous dispersion ( β 2 <0). It is clear that a CS overlapping with the leading (trailing) edge of the phase profile will experience a positive (negative) delay; both scenarios bring the soliton closer to the nearest maximum of the phase profile. At that point, the phase does not vary, hence the drift ceases, and the CSs propagate at the same velocity as the phase peaks: the two do not move further with respect to each other. The phase maxima therefore correspond to stable equilibria, acting as trapping sites for temporal CSs. Significantly, if the phase pattern is adjusted, the CSs will follow. This means that, when multiple CSs are trapped to distinct phase peaks, manipulating the phase of the holding beam enables ultrashort optical CSs to be freely moved in time with respect to each other, that is, to realize a temporal tweezer of light. Experimental setup For experimental demonstration, we use a cavity made up of 100 m of standard optical fibre, corresponding to a cavity roundtrip time t R of 0.48 μs (see Methods). A 1,550 nm wavelength cw laser actively locked near a cavity resonance generates the holding beam. An external electro-optic modulator patterns the phase of the holding beam before its launch into the cavity. The electronic (RF) signal used to drive the modulator is shaped by various components depending on the experiment, as detailed below. Our configuration supports temporal CSs of 2.6 ps duration [18] . As the CSs are far shorter than the cavity roundtrip time, they are truly independent from the boundaries and thousands can in principle fit in the cavity simultaneously. We excite them incoherently through cross-phase modulation between the cw intracavity field and ultrashort pulses picked from the output of a separate mode-locked ‘writing’ laser at a different wavelength [16] , [18] . This writing beam is only used once at the start of each measurement: it is coupled into the cavity using a wavelength-division multiplexer, and the wavelength-division multiplexer also ensures that the writing pulses exit the cavity after a single roundtrip. Once excited, the CSs persist by themselves in the cavity and all the light of the writing laser is blocked. The CS dynamics is monitored by extracting one per cent of the intracavity light at each roundtrip for analysis with a fast photodetector and a real-time digital oscilloscope. Phase modulation trapping We first demonstrate how phase modulation enables robust trapping of temporal CSs. 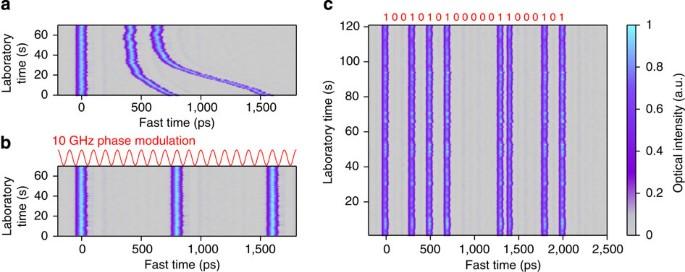Figure 2: Experimental demonstration of cavity soliton trapping. (a) In the absence of any phase modulation on the cavity holding beam, three CSs drift in time due to acoustic-mediated interactions. (b) The interactions are overcome, and the CSs trapped, when applying a sinusoidal phase modulation at 10 GHz (shown in red on top). (c) Phase modulation enables all-optical data storage: A binary-encoded sequence of CSs at 10 Gbit per second is held for two minutes, without distortion. Figure 2a illustrates the behaviour of three temporal CSs, initially excited with an 800 ps relative separation, when propagating in the cavity in the absence of any phase modulation. The colour plot is made up of a vertical concatenation of oscilloscope recordings of the temporal intensity of the light leaving the cavity at each roundtrip, and reveals, from bottom to top, how the three CSs evolve over subsequent roundtrips (the temporal resolution of our photodetector is about 50 ps, hence the figure does not capture how short the 2.6 ps temporal CSs truly are). As can be seen, the temporal separations between the CSs slowly change and the initial bit pattern distorts over time. This occurs because of acoustic-mediated interactions as previously reported [18] . Figure 2: Experimental demonstration of cavity soliton trapping. ( a ) In the absence of any phase modulation on the cavity holding beam, three CSs drift in time due to acoustic-mediated interactions. ( b ) The interactions are overcome, and the CSs trapped, when applying a sinusoidal phase modulation at 10 GHz (shown in red on top). ( c ) Phase modulation enables all-optical data storage: A binary-encoded sequence of CSs at 10 Gbit per second is held for two minutes, without distortion. Full size image In contrast, when repeating the experiment in presence of a 10 GHz sinusoidal phase modulation on the holding beam, Fig. 2b , no sign of interactions or environmental jitter is observed. The temporal CSs are precisely trapped to the modulation. Not only does this result confirm the phase modulation trapping scheme, but it also shows that acoustic interactions do not hinder the potential of temporal CSs for optical buffering applications [16] , [18] . A concrete example of the latter is illustrated in Fig. 2c . Here we show the 10 GHz bit pattern 1001010 1000001 1000101, corresponding to the 7-bit-ASCII representation of ‘JAE,’ successfully buffered as temporal CSs over 2 min (that is, for more than 200 million cavity roundtrips). Demonstration of temporal tweezing Next, we demonstrate the temporal tweezing of trapped CSs. Here, instead of a sinusoidal modulation, we use the configuration depicted in Fig. 3a to generate a reconfigurable phase pattern. A pattern generator produces an electronic signal consisting of quasi-Gaussian pulses with 90 ps duration repeating every 2 ns. That signal is split into two. One of the split signals experiences an additional variable delay Δ τ imparted by an electronic delay line, before it is recombined with the other. The resulting signal is fed to the phase modulator. In this way, we imprint onto the holding beam two identical interleaved sets of phase peaks whose relative temporal separation can be continuously adjusted. 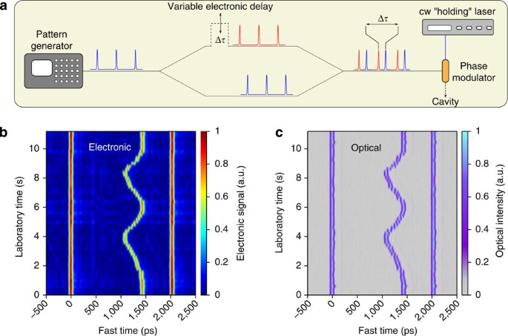Figure 3: Demonstration of the temporal tweezing of temporal CSs. (a) Configuration used to generate an electronic signal consisting of two interleaved periodic sets of 90 ps quasi-Gaussian pulses whose relative delay can be continuously varied. (b) Typical real-time manipulation of the electronic signal and, (c) corresponding identical temporal motion of picosecond optical temporal CSs trapped to the phase peaks. Figure 3: Demonstration of the temporal tweezing of temporal CSs. ( a ) Configuration used to generate an electronic signal consisting of two interleaved periodic sets of 90 ps quasi-Gaussian pulses whose relative delay can be continuously varied. ( b ) Typical real-time manipulation of the electronic signal and, ( c ) corresponding identical temporal motion of picosecond optical temporal CSs trapped to the phase peaks. Full size image Figure 3b illustrates the manipulation of the phase pattern. Using a vertical concatenation of oscilloscope recordings as in Fig. 2 , we show here the electronic signal applied to the phase modulator over time while imposing, by hand, an arbitrary change of the variable delay. The first and the third phase peaks at 0 ps and 2,000 ps, respectively, correspond to consecutive bits of the pattern generator whilst the middle one, initially at 1,400 ps, is the delayed replica of the first. As the delay is continuously varied, the middle phase peak is translated back and forth over a 360 ps range. At the start of this experiment, we also excite three temporal CSs and ensure they are trapped by adjacent peaks of the initial phase pattern. The evolution of the temporal optical intensity profile of these CSs was recorded simultaneously with the electronic phase signal shown in Fig. 3b , and the result is plotted in Fig. 3c . Remarkably, the middle CS tracks precisely, in real time, the changes of the phase pattern, demonstrating a selective dynamic temporal shift—or temporal tweezing—of an ultrashort picosecond light pulse. We must stress that the magnitude of the shift we can impart on our temporal CSs is only limited by the cavity roundtrip time. The 360 ps range demonstrated in Fig. 3c corresponds to 140 pulse widths. While not immediately apparent, the manipulation is also distortionless: the phase modulation does not change the characteristics of the temporal CSs as demonstrated in Supplementary Note 4 and Supplementary Fig. 3 . To further highlight the flexibility of our scheme, Fig. 4 illustrates temporal tweezing in discrete steps. Here manipulation is performed by alternatively switching the phase modulator electronic feed between two distinct (but synchronized) 10 GHz pattern generators ( Fig. 4a ). The patterns are successively reprogrammed at each step to provide independent and simultaneous temporal tweezing of multiple CSs between the 100 ps bit slots of the generators ( Fig. 4b ). A completely reconfigurable optical buffer is a natural outcome of this demonstration. Note that here we have used longer 140 ps electronic pulses, so as to guarantee the trapping of the temporal CSs even after shifting the corresponding phase pulses by 100 ps. 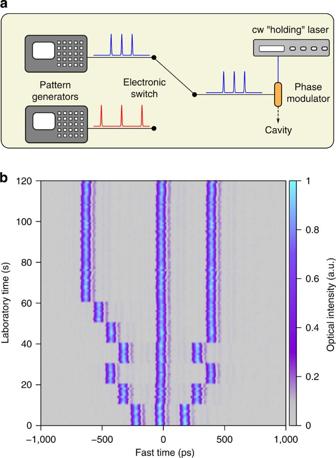Figure 4: Discrete tweezing of temporal CSs. (a) By alternative switching and reprogramming of two synchronized pattern generators, we achieve, (b) discrete simultaneous and independent tweezing of multiple temporal CSs. Figure 4: Discrete tweezing of temporal CSs. ( a ) By alternative switching and reprogramming of two synchronized pattern generators, we achieve, ( b ) discrete simultaneous and independent tweezing of multiple temporal CSs. Full size image Transient attraction dynamics The experimental results above clearly demonstrate how phase modulation of the holding beam permits temporal tweezing of picosecond CSs. These measurements are, however, performed over time scales that do not allow transient CS attraction dynamics to be analysed. In particular, we do not resolve in Fig. 4b the time-scale over which the CSs are attracted to their new position; instead the displacements appear instantaneous. To address this point, we use the configuration depicted in Fig. 5a . A pattern generator is set to generate one 110 ps-long phase pulse per cavity roundtrip time. Before feeding these pulses into the phase modulator, they are sent along one of two different paths set up between two electronic switches, with one of the paths providing a 45 ps extra delay with respect to the other. The experiment is initiated with a single temporal CS trapped to the phase peak. The electronic switches are then abruptly and simultaneously activated, which causes the phase profile to be delayed by 45 ps relative to the CS. That new phase profile is quickly imprinted onto the intracavity field (see Methods for a discussion of this aspect). As a result, the CS finds itself down the phase pulse, approximately where the slope is the steepest, and begins to drift towards the shifted phase peak. We monitor the drift by triggering the real-time oscilloscope from the same signal that controls the electronic switches, and by acquiring a long real-time trace of the CS train that exits the cavity over the roundtrips immediately following the switching. From the time series we then infer the drift rate by direct comparison with a simultaneously measured reference set by the electronic signal driving the phase modulator (see also Methods). 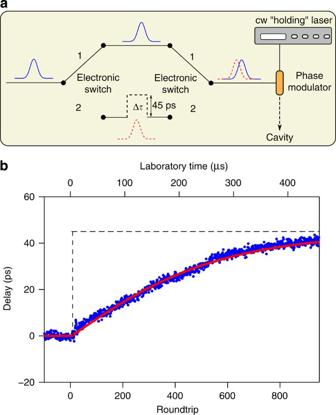Figure 5: Transient phase-modulation attraction dynamics. (a) Electronic circuit allowing a phase pulse trapping a CS to be abruptly delayed by 45 ps. (b) Delay experienced by the CS with respect to its initial position (experiment, blue dots, and theory, red curve) as it is attracted towards the shifted phase peak over 950 roundtrips (or 460 μs). The first 100 roundtrips (with negative numbers) demonstrate the stable trapping of the CS before the switches are activated. The dashed line indicates the maximum of the phase pulse. Figure 5: Transient phase-modulation attraction dynamics. ( a ) Electronic circuit allowing a phase pulse trapping a CS to be abruptly delayed by 45 ps. ( b ) Delay experienced by the CS with respect to its initial position (experiment, blue dots, and theory, red curve) as it is attracted towards the shifted phase peak over 950 roundtrips (or 460 μs). The first 100 roundtrips (with negative numbers) demonstrate the stable trapping of the CS before the switches are activated. The dashed line indicates the maximum of the phase pulse. Full size image Experimental results are shown as blue dots in Fig. 5b . Here we plot the delay of the CS relative to its initial temporal position, with the zero roundtrip point marking the activation of the electronic switches. The first data points (with negative roundtrip numbers) sit stably at 0 ps, and they simply demonstrate the trapping before the phase pulse is temporally shifted. For positive roundtrip numbers we can see the CS being progressively delayed, as it is attracted towards the shifted phase peak, initially with a rate of about 75 fs per roundtrip. Overall, it takes about 400 μs for the CS to settle at the new phase maximum. To compare with theory, we have directly calculated the expected delay accumulated over successive roundtrips by iteratively applying equation (1) with experimental parameters (see Methods). The prediction is shown as the red solid line in Fig. 5b . It is in excellent agreement with experimental observations, confirming our theoretical considerations. Asynchronous phase modulation In the previous experiments, the phase modulation frequency was carefully adjusted to be an integer harmonic of the cavity free-spectral range (FSR). This is not, however, a stringent requirement, and temporal tweezing is reliable even if this condition is not exactly met. In this case, the CS trapping positions are simply slightly offset from the phase maxima, in direct analogy with the offset of particles from the waist of the trapping beam in conventional optical tweezers [37] . This can also be interpreted as a form of frequency locking: the rate at which the CSs recirculate in the cavity is locked to the phase modulation frequency (or to one of its sub-harmonics), instead of being simply equal to the FSR. The theory presented in Supplementary Notes 2 and 3 gives the following condition for the CS trapping position τ CS (measured with respect to a phase maximum): where f PM = N ·FSR+Δ f is the phase modulation frequency and Δ f its offset from the closest harmonic of the FSR. Significantly, a limiting value for the frequency mismatch that the trapping (or frequency locking) process can tolerate can be derived from the above: Here is the maximum of the phase gradient, and φ ( τ ) was assumed time symmetric for brevity. We tested this prediction by trapping a single CS on a sinusoidal phase profile whose frequency was approximately set to 10 GHz ( ∼ 4,819 FSR). We then systematically adjusted the frequency of the modulation so as to scan the offset-frequency Δ f . For each value, we compared the measured photodetector signal with the electronic signal driving the phase modulator, which allowed us to deduce the position of the CS relative to the nearest phase peak (see Methods). Experimental results are shown as the blue dots in Fig. 6 , and are in excellent agreement with the theoretical prediction (red solid line) derived from equation (2). We find an experimental trapping range of Δ f =±534 Hz. Beyond this limit, the CSs are no longer trapped; instead we observe that their relative separation against the RF signal varies from roundtrip-to-roundtrip. This value again matches very well the theoretical limit Δ f max =530 Hz calculated from equation (3) for our experimental conditions, again validating our analysis. 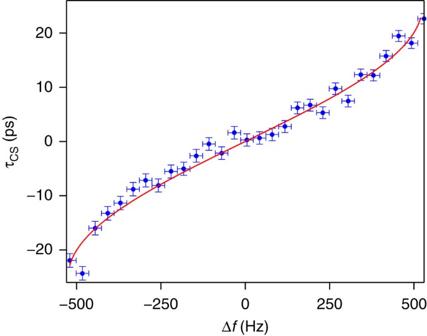Figure 6: Effect of asynchronous phase modulation. The blue dots show experimentally measured temporal position of the stably trapped CS relative to the nearest peak of the sinusoidal phase modulation for a range of frequency mismatch Δf. The red solid curve displays theoretical prediction (see also Methods) and agrees well with the experimental data. Error bars indicate s.d. Figure 6: Effect of asynchronous phase modulation. The blue dots show experimentally measured temporal position of the stably trapped CS relative to the nearest peak of the sinusoidal phase modulation for a range of frequency mismatch Δ f . The red solid curve displays theoretical prediction (see also Methods) and agrees well with the experimental data. Error bars indicate s.d. Full size image The scheme demonstrated in this work enables distortionless trapping and manipulation of picosecond temporal cavity solitons. On the one hand, the trapping mechanism allows for long-range soliton interactions [18] and environmental jitter to be suppressed, which directly permits all-optical buffering for extended periods of time. On the other hand, the ability to dynamically control the pulse positions by manipulating the phase profile of the cavity holding beam renders the buffer fully reconfigurable. All the experimental observations agree completely with theory and numerical simulations (see Supplementary Note 1 and Supplementary Fig. 2 ). Our experiment is not particularly sensitive to any parameters. Of particular significance is the fact that the phase modulation does not have to be accurately synchronized with the cavity FSR, with the observed tolerable frequency mismatch of ±0.5 kHz being sufficiently large to avoid active locking of the phase modulator to the cavity. The speed at which the CS temporal positions can be manipulated is limited by the drift rate [equation (1)]. In our experiments, shifting over a single bit slot in a 10 GHz sequence occurs over approximately 500 μs. Faster manipulation could be obtained by using fibres with larger group velocity dispersion or phase modulation with larger maximum gradient; no attempts have been made at optimization. Miniaturization of the technology could also be possible by harnessing the ability of monolithic microresonators to support temporal CSs [20] . On a more general level, our work illustrates how the unique particle-like characteristics of solitons [38] , [39] can be leveraged to achieve all-optical control of light. Specifically, we have demonstrated arbitrary selective manipulation of the temporal positions of ultrashort optical pulses within a train, with no limitation on the range of time delays over which pulses can be translated. In doing so, we have effectively realized a temporal tweezer for light, in a platform fully compatible with existing fibre-based communication technologies. These results could have significant implications for all-optical information processing. More fundamentally, phase modulation trapping could also be used to probe soliton interactions in a way akin to force microscopy [40] . Basic experimental setup For our experiments, we use a cw pumped passive fibre cavity set-up similar to that used in ref. 18 . The setup is shown in Supplementary Fig. 1 . The cavity is made up of L =100 m of standard single-mode silica optical fibre (Corning SMF-28) with measured group-velocity dispersion β 2 =−21.4 ps 2 km −1 and nonlinearity coefficient γ =1.2 W −1 km −1 at a wavelength of 1,550 nm. The fibre is laid in a ring configuration with a 90/10 input coupler closing the loop. Stimulated Brillouin scattering [41] is prevented with the inclusion in the ring of a fibre isolator with 60 dB extinction. Overall, the cavity has a FSR of 2.075 MHz (or roundtrip time t R =FSR −1 ≃ 0.48 μs) and a finesse =21.5. The cavity is coherently driven with a 1,550 nm-wavelength Koheras AdjustiK E15 distributed-feedback fibre laser (linewidth<1 kHz). The 20 mW cw laser output can be amplified up to 1 W before being coupled into the cavity through the input coupler to act as the ‘holding’ beam. The optical frequency of the laser is actively locked at a set detuning from a cavity resonance with a commercial 100 kHz proportional-integral-derivative controller (SRS SIM960). The error signal of the proportional-integral-derivative controller is simply obtained by comparing the power reflected off the cavity with a reference level. The writing pulses used to excite the temporal CSs via cross-phase modulation are emitted by a 1,532 nm wavelength picosecond mode-locked laser with a 10 GHz repetition rate. Two intensity modulators, one driven by a 10-GHz electronic pattern generator, the other by a gating pulse, are used in sequence to select a single realization of a desired pattern of writing pulses. To trap and manipulate the temporal CSs, the holding beam is phase-modulated using a telecommunications electro-optic phase modulator with a 10-GHz bandwidth. The phase modulator is placed before the cavity input coupler, between the AdjustiK laser and the amplifier. Our experiments are not critically sensitive to the phase modulation amplitude. A peak amplitude of 0.5 rad is typically used, unless specifically mentioned otherwise. The electronic (RF) signal used to drive the modulator is shaped by various RF components depending on the experiment and originates from either a sinusoidal signal generator or an electronic pattern generator. The pulses from our pattern generator are 90-ps long (full width at half maximum), and longer pulses can be obtained when needed with an extra RF filter. In all experiments, the CS dynamics and our temporal manipulations are monitored by extracting one per cent of the intracavity power through an additional fibre tap coupler incorporated into the ring cavity. The extracted light is detected and analysed with a 12.5-GHz amplified PIN photodiode connected to a 40 GSa s −1 real-time oscilloscope. This system has a ∼ 50 ps impulse response which sets the temporal resolution of the fast-time measurements. Oscilloscope acquisition rate The colour plots made up of a vertical concatenation of oscilloscope recordings of the temporal intensity profile of the cavity output have been obtained with a one frame per second acquisition rate for Fig. 2a–c and Fig. 4b , while a rate of five frames per second has been used for Fig. 3b,c . Transient attraction experiment The experimental results shown in Fig. 5 are measured by triggering the real-time oscilloscope from the same TTL signal that controls the electronic switches, and by acquiring a long real-time signal of the CS train that exits the cavity over roundtrips immediately following the switching. Since the oscilloscope has a limited memory depth of 2 million points at the highest sampling rate of 40 GSa s −1 , data can only be acquired about 100 roundtrips at a time. This is not sufficient to reveal the full dynamics. To circumvent this issue, we acquired 10 independent sets of data where the oscilloscope's acquisition window with respect to the TTL trigger is systematically delayed. These sets are then carefully combined so as to obtain a full recording of CS drift dynamics over about 1,000 roundtrips, as shown in Fig. 5 . The delays plotted along the vertical axis of that figure are obtained after fitting Gaussians to the temporal CSs and phase pulses recorded by the oscilloscope at each roundtrip. The uncertainty on those fits results in an error on the delays of σ Delay =1.3 ps (s.d.). The vertical spread of the data visible in Fig. 5 is representative of that error. To obtain the theoretical comparison, we used experimental cavity parameters and inferred the functional form of the phase profile φ ( τ ) by measuring the electronic pulse driving the modulator. It was found to have a smooth Gaussian shape with 110 ps full width at half maximum and an amplitude of 2.7 rad. The theoretical prediction was then obtained by iteratively applying equation (1) over consecutive roundtrips. Note that this calculation assumes that the phase profile trapping the temporal CS is instantaneously delayed on activation of the electronic switches. The time it takes for these switches to operate is very short (about 5 ns) and negligible. However, it takes some more time for the new phase pattern to be imprinted and steady onto the intracavity field, typically a few times the cavity photon lifetime, in our case about ten roundtrips, or 5 μs. As the temporal CS attraction dynamics occurs over about 400 μs, it is clear that this lag can also be neglected in our measurement. The good agreement with theory supports this argument. Asynchronous phase-modulation experiment In experiments examining the effect of asynchronous phase modulation ( Fig. 6 ), the frequency of the sinusoidal electronic signal driving the phase modulator was systematically adjusted in steps of 37.5 Hz. For each value, we simultaneously measured the photodetector signal at the cavity output as well as the electronic signal driving the modulator. The temporal position of the CS relative to the nearest phase maximum was then obtained by comparing the two recorded signals (error analysis was carried out as for Fig. 5 and is depicted by the vertical error bars). Since these signals invariably possess different electrical path lengths, they come with a fixed instrumental temporal delay, preventing direct measurement of the absolute separation. To overcome this, we assume that for perfect synchronisation (Δ f =0) the separation is zero, as predicted by theory, and we justify this assumption a posteriori by the excellent agreement with theoretical predictions seen for all Δ f . To obtain the Δ f=0 reference, we exploit the fact that, for a symmetric phase profile, Δ f=0 occurs midway between the trapping limit frequencies ±Δ f max . They are easy to find since for the CS is not trapped and its separation relative to the RF signal changes from roundtrip-to-roundtrip. The limit frequencies are obtained to within 37.5 Hz which gives rise to a corresponding error on Δ f (horizontal error bars). Since this experiment uses (co)sinusoidal phase modulation, the theoretical prediction for the CS position τ CS can be expressed analytically. Specifically, substituting φ ( τ )= A cos(2 πf PM τ ) into equation (2) we derive: We note that the experimental data shown in Fig. 6 exhibit the expected inverse-sine characteristics. The theoretical prediction shown as the red solid line in this figure has been derived from the above expression, using the experimental phase modulation frequency f PM ≃ 10 GHz and amplitude A =0.19 rad. For the tolerable frequency mismatch, we have , yielding Δ f max =530 Hz. How to cite this article: Jang, J. K. et al. Temporal tweezing of light through the trapping and manipulation of temporal cavity solitons. Nat. Commun. 6:7370 doi: 10.1038/ncomms8370 (2015).